Evidence that asthma is a developmental origin disease influenced by maternal diet and bacterial metabolites Asthma is prevalent in Western countries, and recent explanations have evoked the actions of the gut microbiota. Here we show that feeding mice a high-fibre diet yields a distinctive gut microbiota, which increases the levels of the short-chain fatty acid, acetate. High-fibre or acetate-feeding led to marked suppression of allergic airways disease (AAD, a model for human asthma), by enhancing T-regulatory cell numbers and function. Acetate increases acetylation at the Foxp3 promoter, likely through HDAC9 inhibition. Epigenetic effects of fibre/acetate in adult mice led us to examine the influence of maternal intake of fibre/acetate. High-fibre/acetate feeding of pregnant mice imparts on their adult offspring an inability to develop robust AAD. High fibre/acetate suppresses expression of certain genes in the mouse fetal lung linked to both human asthma and mouse AAD. Thus, diet acting on the gut microbiota profoundly influences airway responses, and may represent an approach to prevent asthma, including during pregnancy. The prevailing explanation for the increase in certain inflammatory conditions such as asthma and allergies has been the hygiene hypothesis [1] , [2] , which proposes that declining family size and improvements in personal hygiene reduce the opportunities for cross-infections in young families. This lack of exposure to infectious agents is thought to result in inappropriate immune regulation, resulting in polarization to Th2 responses. Recently, however, much more attention has focused on diet [3] , [4] , [5] , [6] , or the gut microbiota [7] , [8] , [9] , to explain prevalence of inflammatory diseases particularly in Western countries. Numerous studies have noted a correlation between asthma incidence and obesity [10] , [11] , [12] , [13] . High fat [14] and low fruit and vegetable [15] consumption is correlated with worse asthma outcomes. Furthermore, Western-style fast food increases asthma risk [16] , [17] , [18] , while a Mediterranean diet (high in fish, fruits, nuts and vegetables) protects against wheeze and asthma in childhood [19] . Consumption of fibre is often reduced in severe asthmatics, and associated with increased eosinophilic airway inflammation [20] . Although the above studies suggest that diet or the gut microbiota may influence asthma in humans, the cellular mechanisms that have been evoked to date involve either inadequate immune regulation [21] , or a compromised airway epithelium [22] . It is well documented that asthmatics have fewer T regulatory cells (Tregs), and these are also less functional [21] , [23] . Another view is that asthma is primarily an epithelial disorder [22] , and, in certain susceptible individuals, impaired epithelial barrier function renders the airways vulnerable to various insults, which predispose to asthma. Recently, several groups including our own have outlined mechanisms whereby diet or gut microbial products might affect inflammatory diseases [6] , [24] , Treg biology [25] , [26] , [27] , [28] , dendritic cell (DC) biology [6] or epithelial integrity [29] . Dietary fibre is fermented by colonic commensal bacteria to short-chain fatty acids (SCFAs). SCFAs are anti-inflammatory [24] , promote gut homeostasis [30] and epithelial integrity [4] , [29] , and regulate the size and function of the colonic Treg pool [25] , [26] , [27] . A recent study reported that dietary fibre and the SCFA propionate protected against allergic airway disease (AAD) in mice [6] . This study found that propionate altered DC biology, which affected their ability to promote Th2 responses. SCFAs are known to act via two principal mechanisms: signalling through ‘metabolite-sensing’ G-protein coupled receptors (GPCRs) such as GPR43, GPR41 and GPR109A, and inhibition of histone deacetylases (HDACs) and consequent effects on gene transcription [4] . In one study [31] , HDAC9 proved particularly important in regulating Foxp3-dependent suppression, and optimal Treg function required acetylation of several lysines in the forkhead domain of Foxp3, and this suppressed IL-2 production. Although Foxp3 and its target genes have been implicated mostly in Treg biology [32] , FoxP3 might also be expressed by non-immune cells such as certain epithelia [33] although this topic remains controversial. The important role of Tregs in asthma [21] , coupled with profound effects of SCFAs on Treg biology, prompted us to examine diet and metabolites as a basis for the development of asthma. Here we report that a high-fibre diet promotes a microbiota that produces high levels of SCFAs, particularly acetate, which suppressed the development of AAD in mice. This was dependent on Treg cells, and HDAC9 inhibition by SCFAs was a likely molecular mechanism whereby dietary fibre suppressed AAD, since Hdac9 −/− mice were highly resistant to the development of AAD. Our findings emphasize the importance of diet and bacterial metabolites, over hygiene, to explain asthma. Moreover, in addition to our studies in adult mice, we show that maternal diet and metabolites had profound effects on the developing fetus, by affecting transcription of certain Foxp3 target genes in the lung that have been linked to asthma development. A high-fibre diet shapes gut microbial ecology First, we investigated whether a high-fibre diet alters gut microbial ecology, or produces higher levels of SCFAs in faeces or blood. Faecal pellets were collected after 3 weeks and microbiota composition assessed by 16S sequencing. The diets had marked effects on the composition of the microbiota by both unweighted and weighted UniFrac ( P =2 × 10 −5 , Fig. 1a ). Alpha diversity metrics available in Qiime were compared between the three diets. While there were no significant differences between control and high-fibre, differences were observed between control and no-fibre diet. No-fibre diet had lower Shannon index ( P =0.009), observed species ( P =0.012) and chao1 ( P =0.027) than control. All of the significant metrics with corresponding P values are given in Supplementary Fig. 1 . The diets caused significant perturbations at the phylum level ( Fig. 1b ). Firmicutes dominated with the control diet ( P =8.22 × 10 −6 ; Qiime calculated ANOVA at a phylum level), Bacteroidetes with a high-fibre diet ( P =0.0017) and Proteobacteria with a no-fibre diet ( P =7.49 × 10 −9 ). Interestingly, the high-fibre diet increased ( P =1.53 × 10 −5 and 8.01 × 10 −4 , 58- and 215-fold) two operational taxonomical units (OTUs) of the Bacteroidetes phylum, with 95.0 and 98.5% identity to high-acetate-producing Bacteroides acidifaciens A40(T) strain (EzTaxon database). Differences in abundance were also observed on the family level ( Fig. 1c ). The most representative genera were Clostridium, Bacteroides, Pandoraea and unknown genus of Alphaproteobacteria ( Fig. 1d ). An unknown genus of Alphaproteobacteria appeared only with the high-fibre diet. A massive blooming of Proteobacteria with the no-fibre diet related to the genus Pandoraea , a member of family Burkholderiaceae ( Fig. 1c,d ) with most abundant OTUs from this genera aligning with Pandoraea norimbergensis CCUG 39188(T) strain (97.55 to 99.6% sequence similarity, EzTaxon database). Changes in the microbiota composition prompted us to assess SCFA levels in faeces and serum by NMR spectroscopy. The high-fibre diet increased total SCFA levels in both faeces and serum ( Fig. 1e ). Of the SCFAs, acetate was the most abundant and the high-fibre diet increased acetate in the faeces and serum, whereas the no-fibre diet decreased acetate levels in the serum. In addition, the high-fibre diet increased propionate in the serum, although levels were still very low. Therefore, a high-fibre diet alters the composition of the gut microbiota to produce high levels of SCFAs, leading in particular to high levels of acetate in serum. 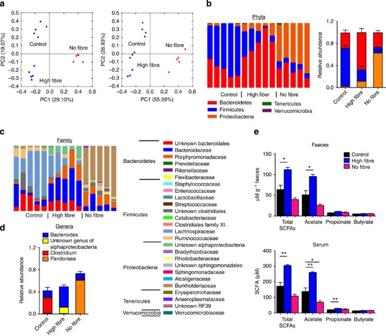Figure 1: High-fibre diet alters the composition of the gut microbiota to produce high levels of acetate. Adult (6 week old female C57Bl6) mice (obtained from the same facility and cohoused for 3 weeks) were provided different diets for 3 weeks then faeces and blood were collected. The composition of the microbiota was significantly different (Anosim, 106permutations) between diets using (a) unweighted (P=2 × 10−5) and weighted UniFrac (P=2 × 10−5) analysis. Control diet (black triangles), high-fibre diet (blue squares), no-fibre diet (red circles). Relative abundance and significantly (ANOVA) different (b) phyla, (c) family and (d) genera. (e) SCFA levels in faeces and serum measured by1H-NMR spectroscopy. Data represent mean+s.e.m.,n=5. Significance is represented by *P<0.05, **P<0.01, Student’st-test. Figure 1: High-fibre diet alters the composition of the gut microbiota to produce high levels of acetate. Adult (6 week old female C57Bl6) mice (obtained from the same facility and cohoused for 3 weeks) were provided different diets for 3 weeks then faeces and blood were collected. The composition of the microbiota was significantly different (Anosim, 10 6 permutations) between diets using ( a ) unweighted ( P =2 × 10 −5 ) and weighted UniFrac ( P =2 × 10 −5 ) analysis. Control diet (black triangles), high-fibre diet (blue squares), no-fibre diet (red circles). Relative abundance and significantly (ANOVA) different ( b ) phyla, ( c ) family and ( d ) genera. ( e ) SCFA levels in faeces and serum measured by 1 H-NMR spectroscopy. Data represent mean+s.e.m., n =5. Significance is represented by * P <0.05, ** P <0.01, Student’s t -test. Full size image High-fibre diet protects against the development of AAD To investigate the immune regulatory effects of diet, and the changes to the microbiota, on AAD, we used the house-dust mite (HDM) model of AAD, which replicates many of the features of human asthma. We fed mice with a control diet, a high-fibre diet (in which the carbohydrates were replaced with high amylose maize resistant starch) or a diet with no-fibre ( Supplementary Table 1 ). All diets contained similar levels of protein, fat and digestible energy, and there were no differences in weight gain over the course of any of the experiments. Mice were provided with the different diets and three weeks later sensitized to HDM intranasally (i.n. day 0, 1 and 2) and challenged i.n. on days 12–15 to induce AAD, which was assessed on day 16 ( Fig. 2a ). In addition, we also administered acetate (200 mM) in the drinking water and assessed the development of AAD. As expected, HDM induced all the characteristic features of AAD: increased total cells and eosinophils in bronchoalveolar lavage fluid (BALF), eosinophils in blood, Th2 cytokine levels and IFN-γ release from mediastinal lymph node (MLN) T cells, IgE levels, lung inflammation, tissue eosinophils, mucous-secreting cells (MSCs) and airway hyper-reactivity (AHR) in terms of airway resistance and dynamic compliance ( Fig. 2b–i ). When the mice consumed the high-fibre diet or acetate in the drinking water, features of AAD failed to develop ( Fig. 2b–i ). Acetate had to be given for at least 3weeks to reduce the development of AAD and acetate still suppressed AAD when administered 3 weeks before sensitization only ( Supplementary Fig. 2 ). Of note, the results were not explained by pH of the acetate solution ( Supplementary Fig. 3 ) and extended to other models of AAD such as ovalbumin (OVA) sensitization ( Supplementary Fig. 4 ). However, acetate did not suppress established AAD ( Supplementary Fig. 5 ), at least using the protocols used here. We also added propionate to the drinking water (200 mM) and found a trend towards lower eosinophil numbers in BALF, decreased IL-13 release from MLN T cells and decreased IgE levels ( Supplementary Fig. 6 ), although these differences did not reach significance. Propionate did result in a small but significant decrease in IL-5 release from MLN T cells. Together these data show that a high-fibre diet and the consumption of acetate, in particular, protects against the development of AAD. 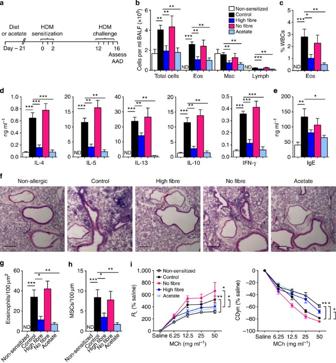Figure 2: The effect of high-fibre diet and acetate on the development of AAD in adult mice. (a) Mice (female C57Bl6) were weaned onto control, high-fibre diet, no-fibre diet, or acetate for 3 weeks and at 6 weeks old sensitized and challenged with HDM. The effect of high-fibre or no-fibre diet on (b) differential cell number in BALF, (c) eosinophils in blood, (d) IL-4, IL-5, IL-13, IL-10 and IFNγ release from MLN T cells, (e) serum IgE, (f) lung histology (scale bar 200 μm), (g) eosinophils in lung tissue, (h) mucous-secreting cells (MSCs) and (i) airway hyper-responsiveness in terms of airway resistance (RL) and dynamic compliance (Cdyn). Data represent mean+s.e.m.,n=8. Significance is represented by *P<0.05, **P<0.01, ***P<0.001, Student’st-test. One representative experiment of three is shown. ND, not detected. Figure 2: The effect of high-fibre diet and acetate on the development of AAD in adult mice. ( a ) Mice (female C57Bl6) were weaned onto control, high-fibre diet, no-fibre diet, or acetate for 3 weeks and at 6 weeks old sensitized and challenged with HDM. The effect of high-fibre or no-fibre diet on ( b ) differential cell number in BALF, ( c ) eosinophils in blood, ( d ) IL-4, IL-5, IL-13, IL-10 and IFNγ release from MLN T cells, ( e ) serum IgE, ( f ) lung histology (scale bar 200 μm), ( g ) eosinophils in lung tissue, ( h ) mucous-secreting cells (MSCs) and ( i ) airway hyper-responsiveness in terms of airway resistance (R L ) and dynamic compliance (Cdyn). Data represent mean+s.e.m., n =8. Significance is represented by * P <0.05, ** P <0.01, *** P <0.001, Student’s t -test. One representative experiment of three is shown. ND, not detected. Full size image Maternal diet suppresses AAD responses in adult offspring High levels of SCFAs could be expected to induce epigenetic modifications, since SCFAs are natural inhibitors of HDACs. We therefor determined whether the protective effect of high fibre diet, or acetate, could extend to the developing fetus. Indeed previous studies have established that maternal exposures may influence asthma symptoms in offspring [34] . Pregnant mice (embryonic age (E)13) were provided with control, high-fibre or no-fibre diet, or acetate in the drinking water ( Fig. 3a ). The offspring were weaned at 3 weeks of age onto the control diet. When the offspring were 6 weeks old, AAD was induced. Strikingly, when the mother consumed the high-fibre diet or acetate, features of AAD failed to develop in the adult (6–8wk old) offspring, as evidenced by a reduction of total cells and eosinophils in BALF, eosinophils in blood, Th2 cytokine and IFN-γ release from MLN T cells, IgE, lung inflammation, tissue eosinophils, MSCs and AHR ( Fig. 3b–i ). Maternal intake of a high-fibre diet or acetate also protected against the development of AAD when the offspring were younger (3 weeks old) or older (16 weeks old) ( Supplementary Fig. 7 ). 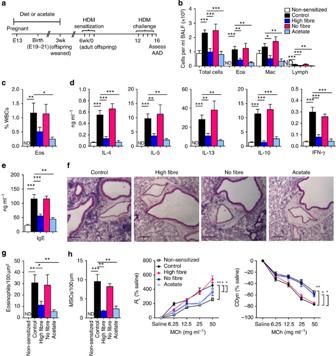Figure 3: The effect of maternal intake of high-fibre diet and acetate on the development of AAD in the offspring. (a) Pregnant mice (E13, C57Bl6) were provided with control, high-fibre diet, no-fibre diet or acetate. Offspring (female C57Bl6) were weaned onto control diet and water at 3 weeks of age and at 6 weeks, sensitized and challenged with HDM. The effect of high-fiber diet or acetate on (b) differential cell number in BALF, (c) eosinophils in blood, (d) IL-4, IL-5, IL-13, IL-10 and IFNγ release from MLN T cells, (e) serum IgE, (f) lung histology (scale bar, 200 μm), (g) eosinophils in lung tissue, (h) mucous-secreting cells (MSCs), and airway hyperresponsiveness in terms of airway resistance (RL) and dynamic compliance (Cdyn). Data represent mean+s.e.m.,n=8. Significance is represented by *P<0.05, **P<0.01, ***P<0.001, Student’st-test. One representative experiment of three is shown. ND, not detected. Figure 3: The effect of maternal intake of high-fibre diet and acetate on the development of AAD in the offspring. ( a ) Pregnant mice (E13, C57Bl6) were provided with control, high-fibre diet, no-fibre diet or acetate. Offspring (female C57Bl6) were weaned onto control diet and water at 3 weeks of age and at 6 weeks, sensitized and challenged with HDM. The effect of high-fiber diet or acetate on ( b ) differential cell number in BALF, ( c ) eosinophils in blood, ( d ) IL-4, IL-5, IL-13, IL-10 and IFNγ release from MLN T cells, ( e ) serum IgE, ( f ) lung histology (scale bar, 200 μm), ( g ) eosinophils in lung tissue, ( h ) mucous-secreting cells (MSCs), and airway hyperresponsiveness in terms of airway resistance (R L ) and dynamic compliance (Cdyn). Data represent mean+s.e.m., n =8. Significance is represented by * P <0.05, ** P <0.01, *** P <0.001, Student’s t -test. One representative experiment of three is shown. ND, not detected. Full size image Effects of maternal diet are mediated in utero Interestingly, we found that consumption of the high-fibre diet or acetate after birth and throughout lactation (birth-3wks) had no effect on the development of AAD in the offspring later in life ( Supplementary Fig. 8 ). In contrast, when mice received high-fibre diet or acetate from E13 until birth only, AAD failed to develop in the offspring ( Fig. 4a–e ). The effect of high-fibre diet and/or acetate may be due to maternal transfer of a specific microbiota to the offspring at birth. We next caesarean-transferred offspring from mice receiving high-fibre diet or acetate to mothers receiving control diet or water ( Fig. 4f ) and found that features of AAD were still markedly reduced in the offspring ( Fig. 4g–j ). Similarly, the same result was seen when the offspring were transferred immediately after birth ( Supplementary Fig. 9 ). However, when offspring were transferred from mothers receiving the control diet or water to mothers that had received high-fibre or acetate, they continued to develop AAD ( Supplementary Fig. 10 ), despite adopting a microbiota more similar to their foster mother ( Supplementary Fig. 11 ). To investigate whether the effect was transferable between mice, we cohoused the offspring from different mothers. Only the mice whose mother received high-fibre diet or acetate failed to develop AAD ( Supplementary Fig. 12 ). Since the microbial transfer was not a key factor in mediating suppression of AAD in the offspring, we investigated whether acetate was being transferred across the placenta to the fetus. It is likely that, levels of acetate in the fetal blood were increased when the mother was on a high-fibre diet or acetate ( Fig. 4k ). Together this data shows that the effects of maternal intake of a high-fibre diet or acetate on AAD are mediated in utero and are independent of transfer of a specific microbiota. 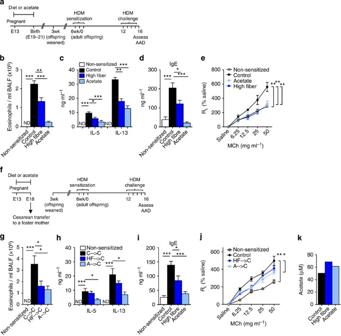Figure 4: Effects of maternal diet or acetate on AAD are mediatedin uteroindependently of microbial transfer. (a) Pregnant mice (E13, C57Bl6) were provided with control, high-fibre diet or acetate. At birth, the control diet or water was provided. Female offsprings were also weaned onto control diet and water at 3 weeks of age and at 6 weeks, sensitized and challenged with HDM. The effect of high-fibre diet or acetate during pregnancy on (b) eosinophil cell number in BALF, (c) IL-5 and IL-13 release from MLN T cells, (d) serum IgE and (e) airway hyperresponsiveness in terms of airway resistance (RL). (f) Pregnant mice (E13) were provided with control, high-fibre diet or acetate. At E18, offspring were caesarean transferred to a foster mother (Balb/c) fed the control diet and water. Female offspring were weaned onto control diet and water at 3 weeks of age and at 6 weeks, sensitized and challenged with HDM. The effect of high-fibre diet or acetate during pregnancy after caesarean transfer on (g) eosinophil cell number in BALF, (h) IL-5 and IL-13 release from MLN T cells, (i) serum IgE and (j) airway hyper-responsiveness in terms of airway resistance (RL). Data represent mean+s.e.m.,n=8. Significance is represented by *P<0.05, **P<0.01, ***P<0.001, Student’st-test. One representative experiment of three is shown. ND= not detected. (k) Serum was collected from offspring (n=35–40 per group) at E18 and acetate levels measured by1H-NMR spectroscopy. Each measurement represents∼35–40 pooled individual blood collections. Figure 4: Effects of maternal diet or acetate on AAD are mediated in utero independently of microbial transfer. ( a ) Pregnant mice (E13, C57Bl6) were provided with control, high-fibre diet or acetate. At birth, the control diet or water was provided. Female offsprings were also weaned onto control diet and water at 3 weeks of age and at 6 weeks, sensitized and challenged with HDM. The effect of high-fibre diet or acetate during pregnancy on ( b ) eosinophil cell number in BALF, ( c ) IL-5 and IL-13 release from MLN T cells, ( d ) serum IgE and ( e ) airway hyperresponsiveness in terms of airway resistance ( R L ). ( f ) Pregnant mice (E13) were provided with control, high-fibre diet or acetate. At E18, offspring were caesarean transferred to a foster mother (Balb/c) fed the control diet and water. Female offspring were weaned onto control diet and water at 3 weeks of age and at 6 weeks, sensitized and challenged with HDM. The effect of high-fibre diet or acetate during pregnancy after caesarean transfer on ( g ) eosinophil cell number in BALF, ( h ) IL-5 and IL-13 release from MLN T cells, ( i ) serum IgE and ( j ) airway hyper-responsiveness in terms of airway resistance ( R L ). Data represent mean+s.e.m., n =8. Significance is represented by * P <0.05, ** P <0.01, *** P <0.001, Student’s t -test. One representative experiment of three is shown. ND= not detected. ( k ) Serum was collected from offspring ( n =35–40 per group) at E18 and acetate levels measured by 1 H-NMR spectroscopy. Each measurement represents ∼ 35–40 pooled individual blood collections. Full size image Evidence that human asthma may associate with maternal diet To investigate the relationship between dietary fibre intake during human pregnancy and SCFA levels, we obtained sera from pregnant women and dietary fibre intake was calculated by a 24 h food recall ( Supplementary Table 2 ). Consistent with previous studies on the relationship between fibre intake and serum acetate levels [35] , we found that high dietary fibre intake during late pregnancy was associated with higher acetate (but not propionate or butyrate) levels in serum ( Fig. 5a ). We next obtained serum from pregnant women and data on the development of respiratory symptoms in their infants, in the first year of life ( Supplementary Table 3 ). Strikingly, maternal acetate (but not propionate or butyrate) levels equal to or above the median were associated with a significant decrease in percentage of infants requiring two or more general practitioner (GP) visits for cough or wheeze and a trend toward reduced parent-reported wheeze ( Fig. 5b ). Furthermore, this association was not observed if the mothers were asthmatic ( Supplementary Fig. 13 , Supplementary Table 4 ). Taken together, these results provide initial evidence for a role of a high-fibre diet and production of acetate in protecting against the development of airway disease in the offspring. 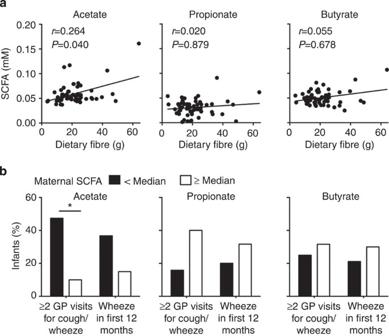Figure 5: SCFA levels and dietary fibre intake in pregnant women, and respiratory symptoms in their offspring. (a) Serum was collected from pregnant women (during late phase pregnancy) and SCFA levels determined by1H-NMR spectroscopy. Dietary fibre was calculated from a 24 h food recall at the same time as serum collection;n=61, Spearman rank correlation. (b) Serum was collected from pregnant women (during late phase pregnancy) and SCFA levels determined by1H-NMR spectroscopy. Percentage of offspring (infants) with ≥2 general practitioner (GP) visits for cough/wheeze and with parent-reported wheeze in the first 12 months was recorded. Solid bars represent mothers with SCFA <median (acetate=0.05315, mM, propionate=0.03083, mM, butyrate=0.03385, mM) open bars represent mothers with SCFA ≥median,n=40, *P<0.05,χ2-test. Figure 5: SCFA levels and dietary fibre intake in pregnant women, and respiratory symptoms in their offspring. ( a ) Serum was collected from pregnant women (during late phase pregnancy) and SCFA levels determined by 1 H-NMR spectroscopy. Dietary fibre was calculated from a 24 h food recall at the same time as serum collection; n =61, Spearman rank correlation. ( b ) Serum was collected from pregnant women (during late phase pregnancy) and SCFA levels determined by 1 H-NMR spectroscopy. Percentage of offspring (infants) with ≥2 general practitioner (GP) visits for cough/wheeze and with parent-reported wheeze in the first 12 months was recorded. Solid bars represent mothers with SCFA <median (acetate=0.05315, mM, propionate=0.03083, mM, butyrate=0.03385, mM) open bars represent mothers with SCFA ≥median, n =40, * P <0.05, χ 2 -test. Full size image Hdac9 −/− mice are protected against AAD We next sought to understand mechanisms whereby diet and metabolites affected AAD, in both adults, and in offspring exposed to high-fibre/acetate in utero . We have demonstrated previously that the metabolite-sensing receptor GPR43 plays a role in the regulation of inflammatory responses, including OVA-induced AAD [24] . Trompette et al. [6] likewise established a role for another SCFA-sensing receptor, GPR41, in the regulation of AAD. Both GPR43 and GPR41 bind acetate, as well as other SCFAs with various affinities. High-fibre diet and acetate still suppressed AAD in Gpr43 -deficient mice ( Supplementary Fig. 14 ), suggesting that signalling via GPR43 was not required for suppression of AAD. This result was a deviation from our previous study [24] and presumably relates to animal house differences or different AAD models. Regardless, this prompted us to explore a role for HDACs, as SCFAs are known inhibitors of HDAC activity. Indeed, cells from whole-lung of acetate-treated adult mice had reduced HDAC activity ( Fig. 6a ). However, acetate had no effect on HDAC activity in the offspring ( Fig. 6a ). It is unknown which HDAC class acetate affects specifically, although HDAC9 has been strongly implicated in the control of Treg biology [31] . In support of this, we found that Hdac9 −/− mice were highly resistant to the development of AAD ( Fig. 6b–e ). Furthermore, when Hdac9 −/− females were crossed with WT males, the Hdac9 +/− offspring were protected against the development of AAD ( Fig. 6f ). Although indirect, this highlights the possibility that acetate may inhibit HDAC9, as there are similar effects of acetate-feeding, and HDAC9 deficiency, on AAD. 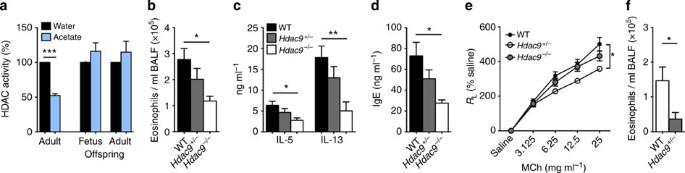Figure 6: The effect of acetate on HDAC activity in the lung, and the development of AAD inHdac9−/−versus WT (C57Bl6, female) mice. (a) HDAC activity in the whole lung (n=6). Development of AAD inHdac9−/−versus WT mice in terms of (b) eosinophil cell number in BALF, (c) IL-5 and IL-13 release from MLN T cells, (d) serum IgE and (e) airway hyperresponsiveness in terms of airway resistance (RL). (f) Eosinophils in BALF in Hdac9+/−offspring from Hdac9−/−females crossed with WT males, in the HDM AAD model. Data represent mean+s.e.m.,n=8. Significance is represented by *P<0.05, **P<0.01, ***P<0.001, Student’st-test. One representative experiment of three is shown. Figure 6: The effect of acetate on HDAC activity in the lung, and the development of AAD in Hdac9 −/− versus WT (C57Bl6, female) mice. ( a ) HDAC activity in the whole lung ( n =6). Development of AAD in Hdac9 −/− versus WT mice in terms of ( b ) eosinophil cell number in BALF, ( c ) IL-5 and IL-13 release from MLN T cells, ( d ) serum IgE and ( e ) airway hyperresponsiveness in terms of airway resistance ( R L ). ( f ) Eosinophils in BALF in Hdac9 +/− offspring from Hdac9 −/− females crossed with WT males, in the HDM AAD model. Data represent mean+s.e.m., n =8. Significance is represented by * P <0.05, ** P <0.01, *** P <0.001, Student’s t -test. One representative experiment of three is shown. Full size image Acetate promotes Treg suppression of AAD HDAC inhibition is known to induce Treg cells [31] . We assessed acetylation at the Foxp3 promoter region and found that acetate increased acetylation at H4 in both the adult and the offspring ( Fig. 7a ), which depicts a ‘primed’ Foxp3 state. Indeed, Foxp3 was expressed at higher levels in whole-lung of acetate-treated mice, both adults and offspring, but only when AAD was induced ( Fig. 7b ). This extended to an increase in the percentage and number of Tregs in peripheral lymph nodes in adult and offspring, when AAD was induced ( Fig. 7c ). Furthermore, the Tregs from mice receiving acetate were more suppressive on a per cell basis ( Fig. 7d ). To confirm the importance of Tregs, we next employed anti-CD25 to deplete Tregs, and showed that Tregs were required for acetate-mediated suppression of AAD in adult mice ( Fig. 7e–h ). Furthermore, to address whether the inheritable suppression of AAD induced by acetate involves Tregs and can be recapitulated in young mice, we administered anti-CD25 to 3-week-old offspring from mothers given acetate during pregnancy and induced AAD. Acetate administered to pregnant mothers suppressed AAD in young offspring, and this was at least partially dependent on Treg cells ( Fig. 7i ). Therefore, acetate promotes acetylation at Foxp3, which promotes Tregs that are highly suppressive and required for suppression of AAD in both young and adult mice. 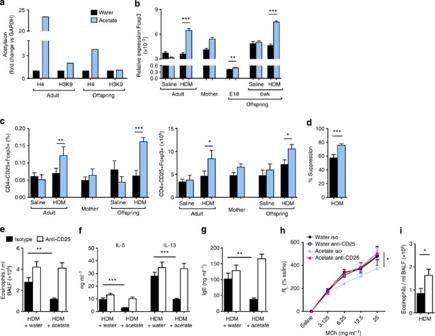Figure 7: Priming of Foxp3, Foxp3 expression and Treg in acetate-mediated suppression of AAD. (a) Acetylation of histones at the Foxp3 promoter (adult=acetate from day -21 to end of model, offspring=acetate by mother D12-weaning). (b) Foxp3 expression in the lung. (c) Percentage and number of Treg cells in the lung. (d) Effect of acetate on Treg suppressive capacity (Treg isolated from the spleen of mice receiving water or acetate). The effect of anti-CD25 mediated Treg depletion on acetate mediated suppression of AAD in terms of (e) eosinophil cell number in BALF, (f) IL-5 and IL-13 release from MLN T cells, (g) serum IgE and (h) airway hyperresponsiveness in terms of airway resistance (RL). (i) AAD and the effect of anti-CD25 mediated Treg depletion in 3-week-old female offspring from mothers (C57Bl6) fed acetate, in terms of eosinophil cell number in BALF. Data represent mean+s.e.m.,n=8. Significance is represented by *P<0.05, **P<0.01, ***P<0.001, Student’st-test. One representative experiment of three is shown. Figure 7: Priming of Foxp3, Foxp3 expression and Treg in acetate-mediated suppression of AAD. ( a ) Acetylation of histones at the Foxp3 promoter (adult=acetate from day -21 to end of model, offspring=acetate by mother D12-weaning). ( b ) Foxp3 expression in the lung. ( c ) Percentage and number of Treg cells in the lung. ( d ) Effect of acetate on Treg suppressive capacity (Treg isolated from the spleen of mice receiving water or acetate). The effect of anti-CD25 mediated Treg depletion on acetate mediated suppression of AAD in terms of ( e ) eosinophil cell number in BALF, ( f ) IL-5 and IL-13 release from MLN T cells, ( g ) serum IgE and ( h ) airway hyperresponsiveness in terms of airway resistance (R L ). ( i ) AAD and the effect of anti-CD25 mediated Treg depletion in 3-week-old female offspring from mothers (C57Bl6) fed acetate, in terms of eosinophil cell number in BALF. Data represent mean+s.e.m., n =8. Significance is represented by * P <0.05, ** P <0.01, *** P <0.001, Student’s t -test. One representative experiment of three is shown. Full size image High-fibre/acetate promote gene regulation in fetal lung Foxp3 is expressed by certain epithelia in the lung [33] . As acetylation at the Foxp3 promoter was altered in the offspring when the mother received acetate in the drinking water, we speculated that gene expression in the lung may be affected by metabolites in utero . Using microarray, we identified 23 genes, some of which were highly differentially expressed in the lung of E21 fetuses from high-fibre fed mothers versus control groups, and 20 differentially expressed genes between acetate and control groups ( Supplementary Fig. 15 , Supplementary Table 5 ). The majority of genes identified were downregulated, which included the genes with the highest fold-change. Molecular network analysis indicated that putative targets for the effects of both high-fibre and acetate were principally involved in embryonic and organ development, cardiovascular disease, developmental disorders and others ( Supplementary Tables 6–8 ). As both high-fibre and acetate suppressed the development of AAD, we focused on genes that associated with both groups ( Fig. 8a , Supplementary Table 5 ). Three genes Nppa, Ankrd1 and Pln were markedly downregulated in the lungs of both the high-fibre and acetate-fed groups, versus control-fed mice, and recorded the highest fold-changes ( Fig. 8b , Supplementary Table 5 ). These genes (and Nppb ) are co-regulated ( Supplementary Fig. 16 ), and their downregulation was confirmed using RT-qPCR ( Fig. 8c ). Nppa encodes for atrial natriuretic peptide (ANP), a molecule mostly associated with heart function, but which also has immune-modifying effects [36] . We confirmed lower ANP protein in the lungs by western blot ( Fig. 8d ). Moreover, Nppa transcripts remained downregulated when the offspring were adults ( Fig. 8e ) suggestive of a sustained epigenetic modification. We then investigated whether HDAC9 was involved in regulation of ANP. Interestingly, network analysis predicted that HDAC9 was an inhibited upstream regulator ( Supplementary Table 6 ), which reiterates our findings in Hdac9 −/− mice ( Fig. 6b–e ). Indeed, the whole lung of Hdac9 −/− mice expressed very low amounts of ANP compared with WT mice ( Fig. 8f ). Therefore, acetate-mediated inhibition of HDAC9 is likely to account for the downregulation of ANP. We then investigated whether Foxp3 was involved in the downregulation of Nppa. Indeed, Nppa-bound Foxp3 was detected at higher levels when the mice received acetate ( Fig. 8g ), thereby demonstrating that Foxp3 binds directly to the Nppa promoter region, which contains six putative binding sites ( Supplementary Fig. 17 ). Together these data demonstrate that acetate alters gene expression in the fetal lung, including downregulation of Nppa , which involves inhibition of HDACs (likely HDAC9) and Foxp3 binding upstream of Nppa to suppress ANP production. 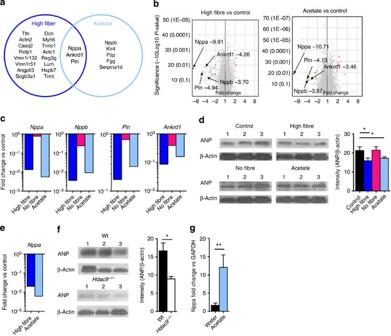Figure 8: The effect of maternal diet and acetate on gene expression in the fetal lung. (a) Venn diagram representation of gene expression in female fetal lung from mothers (C57Bl6) receiving high-fibre diet or acetate versus control, >2-fold change,P<0.05,n=4. (b) Gene expression profile in fetal lungs by volcano plot of offspring from mother receiving high-fibre diet versus control and mother receiving acetate versus control. Fold change <2 (green dots) and >2 (red dots) whereP<0.05 (P>0.05 grey dots),n=4. (c) The effect of diets and acetate on (c)Nppa, Nppb, PlnandAnkrd1gene expression and (d) ANP in fetal lung, assessed by western blot. The effect of diets and acetate on (e)Nppagene expression in adult lung, and (f) ANP levels in whole lungs ofHdac9−/−versus WT mice. (g) Foxp3 was immunoprecipitated from splenocytes and screened forNppagene expression versus GAPDH by RT-PCR. Data represent mean+s.e.m.,n=3, *P<0.05, Student’st-test. One representative experiment of three is shown. Throughout this figure, blue bars=high-fibre fed, red bars=no-fibre fed, and green bars=acetate-fed. Figure 8: The effect of maternal diet and acetate on gene expression in the fetal lung. ( a ) Venn diagram representation of gene expression in female fetal lung from mothers (C57Bl6) receiving high-fibre diet or acetate versus control, >2-fold change, P <0.05, n =4. ( b ) Gene expression profile in fetal lungs by volcano plot of offspring from mother receiving high-fibre diet versus control and mother receiving acetate versus control. Fold change <2 (green dots) and >2 (red dots) where P <0.05 ( P >0.05 grey dots), n =4. ( c ) The effect of diets and acetate on ( c ) Nppa, Nppb, Pln and Ankrd1 gene expression and ( d ) ANP in fetal lung, assessed by western blot. The effect of diets and acetate on ( e ) Nppa gene expression in adult lung, and ( f ) ANP levels in whole lungs of Hdac9 −/− versus WT mice. ( g ) Foxp3 was immunoprecipitated from splenocytes and screened for Nppa gene expression versus GAPDH by RT-PCR. Data represent mean+s.e.m., n =3, * P <0.05, Student’s t -test. One representative experiment of three is shown. Throughout this figure, blue bars=high-fibre fed, red bars=no-fibre fed, and green bars=acetate-fed. Full size image This study highlights the importance of a high-fibre diet and acetate in priming Foxp3-mediated protection against the development of asthma. A general scheme for this model is summarized in Fig. 9 . We showed that a high-fibre diet altered the composition of the microbiota, increased SCFA production (particularly acetate) and protected against the development of AAD in adult mice. One of the main cellular mechanisms related to acetate effects on Treg cells, particularly HDAC inhibition and epigenetic modification of the Foxp3 promoter. As acetate crosses the placenta, and previous studies had suggested a role for maternal influences on asthma development in offspring, we assessed effects of maternal diet during fetal development. These studies indicated an additional ‘developmental origin’ to asthma, whereby in utero effects of maternal diet shape immune responses in the airways of offspring later in life. This also involved Treg biology, but also likely involves Foxp3-regulated genes in other cell types such as epithelia. 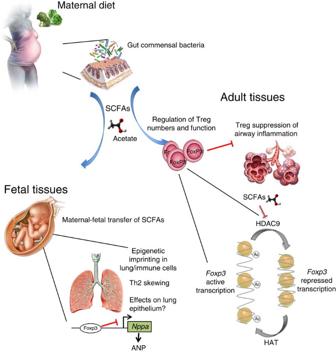Figure 9: Schematic representation of mechanism underlying the effect of maternal fibre intake on the development of asthma, both in the adult, and in offspring. Fibre consumption leads to changes in the microbiota and SCFA production. Acetate enters the bloodstream and inhibits HDACs, leading to transcription of Foxp3. Foxp3 promotes Treg numbers and function, which suppress airway inflammation. During pregnancy, SCFAs such as acetate are capable of crossing the placenta, and influencing gene expression in the fetal lung, such asNppa, which encodes ANP, a molecule implicated in epithelial biology and immune regulation. It is also likely that maternally transferred acetate affects Treg biology in the fetus. Figure 9: Schematic representation of mechanism underlying the effect of maternal fibre intake on the development of asthma, both in the adult, and in offspring. Fibre consumption leads to changes in the microbiota and SCFA production. Acetate enters the bloodstream and inhibits HDACs, leading to transcription of Foxp3. Foxp3 promotes Treg numbers and function, which suppress airway inflammation. During pregnancy, SCFAs such as acetate are capable of crossing the placenta, and influencing gene expression in the fetal lung, such as Nppa , which encodes ANP, a molecule implicated in epithelial biology and immune regulation. It is also likely that maternally transferred acetate affects Treg biology in the fetus. Full size image Many studies now implicate an altered gut microbiota for the pathogenesis of various diseases. Gut microbiota composition relates to diet [9] , [37] ; hence, a causative factor for asthma susceptibility may be insufficient consumption of dietary fibre, although antibiotic use could be an additional factor. A Western diet-shaped gut microbiota may produce lower amounts of SCFAs [38] . In our study, change in dietary fibre consumption led to clear variations in the microbiota, evidenced by distinct population clustering in principle component analysis. Further analysis revealed a small decrease in microbial diversity when mice were fed a no-fibre diet, which parallels associations between Western and low-fibre diets and reduced diversity in human population studies [38] , [39] . However, more marked changes were observed in phylogenetic specifications. Our data in mice showed that high-fibre diet increased Bacteroidetes and decreased Firmicutes, which parallels findings in humans [38] . No-fibre diet enriched Proteobacteria, which has been associated with Western diets and disease states [38] , [40] , [41] . On the family level, high-fibre diet supported the outgrowth of Bacteroidaceae, as reported elsewhere [6] . This family contains particularly high-SCFA-producing bacteria such as Bacteroides acidifaciens, of which similar species were detected in our analysis. Bacteroides have been associated with increases in Foxp3 expression among CD4+ T cells [28] . Altogether our study shows that a high-fibre diet, which was effective at preventing robust AAD in mice, supports a microbiota containing a high abundance of regulatory and non-pathogenic bacteria, which produce high levels of immunoregulatory products such as SCFAs. We have shown previously that acetate feeding suppressed AAD, implicating a role for fibre. Recently, Trompette et al. [6] showed similar findings on the role of dietary fibre. However, we establish a distinct cellular and molecular mechanism: acetate effects on Treg biology. This fits with the established role of SCFAs in regulating HDAC activity, and the important role of Tregs in asthma pathogenesis [21] . A clear result from the present study was the important role of HDAC9 for development of AAD. We showed that Hdac9 −/− mice were resistant to the development of AAD, suggesting that HDAC9 may in part be involved in acetate-mediated suppression of AAD. Indeed, Hdac9 −/− mice have increased numbers of Tregs [31] , which are known to suppress the development of AAD [42] . Furthermore, higher levels of Hdac9 have been reported in human asthmatics [43] . More specific analysis revealed that the Foxp3 promoter region was highly acetylated at H4 and H3K9. Foxp3 activity is regulated by reversible acetylation, and these acetylation patterns are an indicator of a primed transcriptional state [44] , [45] . Indeed, acetylation levels correlated with Foxp3 gene expression and Tregs number, when AAD was induced, presumably because Tregs are required to prevent inflammation. We speculate that inadequate Treg immune regulation in individuals that consume insufficient quantities of fibre may lead to inappropriate immune responses to airborne and gut-encountered allergens. Such a defect may be additive to other pathways relating to diet or gut microbiota, and asthma pathogenesis. A striking finding from this study was the ability of maternal diet to shape airway responses in offspring, later in life. On top of the influences that determine airway responses during adulthood, this adds another dimension to the aetiology of asthma. However, molecular and cellular pathways likely overlap. Acetate is the likely mediator of this developmental effect, as acetate in drinking water also yielded similar effects, and acetate is the predominant metabolite produced from fibre by gut bacteria. Acetate is also the main SCFA distributed throughout the body, including to the developing fetus. For instance the concentrations of acetate, butyrate and propionate in the lower colon range from 20 to 40 mM, yet in the blood butyrate and propionate are usually <5 uM, while acetate is 50–100 uM. There is a large body of evidence for epigenetic influences in utero , which manifest later in life [46] particularly with regard to obesity, diabetes and cardiovascular disease. The actions of HDACs are one of the main epigenetic mechanisms for the regulation of gene transcription. We also provided preliminary evidence that a developmental origin of asthma could be extended to humans. Our data showed a positive correlation between dietary fibre intake and acetate levels in serum. This finding supports other studies that show high-fibre diet correlates with high SCFA levels [38] . We found that high-acetate levels in pregnant individuals correlated with reduced GP visits for cough and wheeze per year and wheeze in the first 12 months for their offspring. These features are some of the most significant predictors for the subsequent development of asthma in later life [47] , [48] . Future analysis, when the children are older, will determine whether these children do indeed go on to develop asthma. Another mechanism whereby bacterial metabolites may influence asthma susceptibility is through effects on cell types in the lung, other than Tregs. This fits with evidence for an epithelial cell contribution to asthma pathogenesis. High-fibre/acetate consumption during pregnancy led to marked downregulation of Nppa transcripts in the lung. The Nppa gene in humans has known polymorphisms that are associated with asthma, with SNPs in the minor allele conferring protection [49] , [50] . How these SNPs affect the transcription of Nppa and subsequent function and level of expression of ANP remains to be determined. ANP binding to its receptors in the airways has been implicated in causing persistent pro-inflammatory effects. In one study, isatin, an endogenous inhibitor of ANP receptor (NPRA) signalling and expression, inhibited airway inflammation in a mouse model of allergic asthma. Leukocyte infiltration to the airways, and airway hyper-reactivity were markedly suppressed by blocking ANP signalling [51] . Receptors for ANP are highly expressed in the lung tissue, including the lung epithelium. Mice deficient in NPRA are resistant to methacholine-induced bronchoconstriction [52] . Another report found that ANP polarizes human DCs towards a Th2-promoting phenotype [36] . Therefore, it is likely that inhibition of Nppa transcript expression and the subsequent effect on ANP protein levels is consistent with protection against AAD. Our finding that Hdac9 −/− mice show very low expression of ANP strengthens this conclusion. Furthermore, we found that acetate increased Nppa-bound Foxp3, demonstrating that Foxp3 binds directly to the Nppa promoter region. Acetate-induced Foxp3 binding to Nppa implicates Foxp3 not only in Treg induction but also direct silencing of certain genes. Indeed, Foxp3 binding to promoter regions has been associated with gene silencing [53] . It will be important to determine the precise role of Foxp3 in gene regulation in various cell types other than Tregs, such as macrophages/DCs or epithelial cells. Deficiency of acetate/SCFAs and consequent higher ANP production by DCs or epithelial cells may be one mechanism responsible for skewing T-cell responses to Th2. The fact that acetate and dietary fibre had such a profound effect on gene expression in the fetal lung may relate to the developmental state of cells, and the fact they have yet to be ‘locked in’ to a gene expression programme [54] . Thus, environmental effects that influence epigenetic mechanisms may be particularly prominent in the developing fetus. In summary, our findings show that high-fibre diet via the production of acetate primes Foxp3-mediated protection against the development of asthma. These findings align with the current understanding that Tregs are critical in maintaining immune regulation in asthma [21] . These findings potentially explain one aspect of the ‘inheritance’ of asthma, via diet and epigenetic effects. Furthermore, our data link known gene associations with the development of asthma. Our data may relate to other associations such as the low incidence of asthma in children growing up on a farm [55] , which we speculate may relate to dietary differences between rural and urban settings, or may relate to microbes encountered in the farm environment that are geared for high SCFA production (that is, faeces from livestock that mostly digest fibre). Other organs and disease processes may well be affected by maternal diet and epigenetic effects, such as cardiovascular disease [56] and may involve similar pathways—microbiota-mediated production of SCFAs, acetylation leading to Foxp3 expression and regulation of target genes within Treg cells, or other Foxp3-expressing cells. Animals Female C57Bl6 and BALB/c mice were obtained from the Monash Animal Research Platform, Monash University. Gpr43 −/− and Hdac9 −/− mice were bred and maintained at the Monash Animal Research Platform. All mice were maintained under specific pathogen-free and controlled environmental conditions and randomly allocated to groups. All procedures were approved by the Animal Ethics Committee of Monash University. Diet and SCFAs Diets used were ‘Control’ (8720310), ‘High fibre’ (SF11-025) and ‘No fibre’ (SF09-028) (Specialty feeds, Perth, Australia; see Supplementary Table S1 for nutritional parameters) and were refreshed three times per week. Acetate or propionate (200 mM, except where indicated) was dissolves into the drinking water and refreshed three times per week. SCFA levels were determined by 1 H-NMR spectroscopy [57] . Bacteria DNA sequencing and bioinformatics DNA was extracted in accordance with method of Yu and Morrison [58] . In brief, DNA was extracted and purified using QIAamp DNA stool mini kit (Qiagen) and amplified using primers selected to cover V1-V3 region of bacterial 16s rRNA gene. Sequencing of 16s RNA gene amplicons was performed with Roche/454 FLX Genome Sequencer using Titanium chemistry and manufacturer’s protocols and kits. Data analysis was done using PyroBayes [59] , Pintail [60] and Acacia [61] for pre-processing, and final analysis using Qiime v1.6.0 (ref. 62 ) with quality trimming settings: sequence lengths of 300–600 bases, no ambiguous sequences and a maximum of 6 homopolymer bases. Data have been deposited into the metagenomic database MG-RAST, ID 12662. Models of AAD Mice were sensitized to HDM ( Dermatophagoides pteronyssinus ) extract (i.n. ; day 0, 1 and 2; 50 μg; Greer Labs, Lenoir, NC) in sterile saline (50 μl) and challenged with HDM (i.n. ; day 14–17; 5 μg in 50 μl saline) under isofluorane anaesthesia. Where indicated mice were sensitized to OVA (i.p. ; day 0 and 7; 50 μg; Sigma-Aldrich, St Louis, MO) with Rehydrogel (1 mg; Reheis, Berkeley Heights, NJ) in sterile saline and challenged (i.n. ; day 12–15; 10 μg in 50 μl saline). To recapitulate established disease, mice received HDM (i.n. ; day 0, 1 and 2; 50 μg) followed by two sets of challenges (days 11–13 and 33–34) [64] . Where indicated, mice received an anti-CD25 antibody (i.p; day -3; 100 μg, PC61). Assessment of AAD BALF and blood cell counts were performed [64] . Cytokine release from MLN and serum IgE was assessed by ELISA. Single-cell suspensions were prepared from MLNs by pushing through 70-μm sieves. A total of 1 × 10 6 cells per well in 96-well U-bottomed plates were cultured in RPMI media supplemented with 10% FCS, HEPES (20 mM), penicillin/streptomycin (10 μg ml −1 ), L -glutamine (2 mM), 2-mercaptoethanol (50 μM), sodium pyruvate (1 mM). Cells were stimulated with HDM (20 μg ml −1 ) and cultured for 96 h (37 °C, 5% CO 2 ). Lungs were perfused, inflated, fixed, embedded, sectioned and stained to enumerate tissue eosinophils (H&E) and MSCs [23] . AHR was assessed as per the manufacturer’s instructions [63] , [64] . The investigator was blinded to experimental groups. Serum acetate from mothers STUDY 1. Serum samples were collected from n =40 pregnant women without asthma, who were participating in a prospective cohort study of viral infection in pregnancy at the John Hunter Hospital, Newcastle between 2007 and 2009 (ref. 65 ). Samples were collected at a median gestational age of 37.6 weeks (interquartile range: 36.6, 38.4 weeks). Infants of these mothers were prospectively followed to 12 months of age [66] and a validated parent completed questionnaire [67] on respiratory health, family medical history, immunizations and infant feeding was completed. STUDY 2. Serum samples were collected from n =61 pregnant women who were participating in a prospective cohort study at the John Hunter Hospital, Newcastle between 2004 and 2006 (refs 65 , 68 ). Samples were collected at a median gestational age of 36 weeks. At this time, women also completed a 24 h food recall. Data were analysed using the Foodworks database (Xyris, Brisbane) [68] . All procedures were approved and patient consent was obtained. HDAC activity Nuclear extracts were isolated using an extraction kit (Abcam) and HDAC activity assays (BioVision) were performed as per the manufacturer’s instructions. Chromatin immunoprecipitation ChIP was performed as per the manufacturer’s instructions. In brief, CD4+Foxp3 cells were fixed in 0.6% paraformaldehyde, washed with PBS then lysed in NP-40 lysis buffer (0.5% NP-40, 10 mM Tris-HCL at pH 7.4, 10 mM NaCl, 10 mM MgCl 2 and protease inhibitors) followed by SDS lysis buffer (1% SDS, 10 mM EDTA, 50 mM Tris-HCl at pH 8.1 and protease inhibitors). Sonicated chromatin product was diluted in 1% Tritox X-100, 20 mM Tris-HCl at pH 8.0, 150 mM NaCl, 2 mM EDTA and protease inhibitors then pre-cleared with Protein A/G–Sepharose and salmon sperm. ChIP was performed with Anti-acetyl-Histone H3 (Lys9) and Anti-hyperacetylated Histone H4 (Penta) Antibody (Millipore, USA). Chromatin was isolated with Protein A/G–Sepharose and washed with low-salt buffer (0.1% SDS, 1% Triton X-100, 20 mM Tris-HCl at pH 8.1, 150 mM NaCl and 2 mM EDTA), high-salt buffer (0.1% SDS, 1% Triton X-100, 20 mM Tris-HCl at pH 8.1, 500 mM NaCl and 2 mM EDTA) and diluted in LiCl buffer (0.5% NP-40, 0.5% Deoxycholate, 10 mM Tris-HCl at pH 8.1, 1 mM EDTA and 0.25 M LiCl). DNA was eluted in elution buffer (1% SDS and 100 mM NaHCO 3 ), de-crosslinked by high-salt treatment (200 mM NaCl) at 65 °C and treated with proteinase K (40 μg ml −1 proteinase K, 10 mM EDTA, 40 mM Tris-HCl at pH 8.1) at 50 °C. Isolated DNA was subject to qPCR using primers specific for GAPDH (F 5′-CTG CAG TAC TGT GGG GAG GT-3′, R 5′-CAA AGG CGG AGT TAC CAG AG-3′), Foxp3 promoter (F 5′-CTG AGG TTT GGA GCA GAA GGA, R 5′-GAG GCA GGT AGA GAC AGC ATT G-3′). Nppa promoter (F 5′-TCT TCT GCT GGC TCC TCA CT-3′, R 5′-GCA CGA TCT GAT GTT TGC TG-3′). Treg assessment A total of 1 × 10 6 cells per well in 96-well U-bottomed plates were stained for CD4, CD25 and Foxp3 using the eBioscience perm kit as per manufacturer’s instructions and analysed by flow cytometry. For suppression assays CD4+Foxp3GFP+ and CD4+Foxp3GFP cells were isolated by FACS (>95% pure). CD4+Foxp3GFP cells (5 × 10 4 ) and varying numbers of CD4+Foxp3GFP+ cells were cultured in RPMI (200 μl, 10% fetal calf serum; 72 h, 37 °C) with anti-CD28 (1 μg ml −1 ; BD Pharmingen) and plate bound anti-CD3 (1 μg ml −1 ). Cells were pulsed for the final 18 h of culture with [ 3 H] thymidine (Amersham International, UK) and enumerated using a microbeta counter. Gene array and RT-PCR Cells were lysed in Trizol and RNA extracted as per manufacturer’s instructions (Sigma). Gene array was carried out using Affymetrix (Ramacoitti Centre, Sydney) including analysis by Affymetrix Transcription Analysis Console (TAC) 2.0 software. For RT-PCR, RNA was reverse transcribed into cDNA and gene expression determined by SYBR Green (Sigma) incorporation relative to the house keeping gene rpl13 (F 5′-ATC CCT CCA CCC TAT GAC AA-3′, R 5′-GCC CCA GGT AAG CAA ACT T-3′). Foxp3 (F 5′-ACT CGC ATG TTC GCC TAC TT-3′, R 5′-AGG GAT TGG AGC ACT TGT TG-3′), Ankrd1 (F 5′-TGC GAT GAG TAT AAA CGG ACG-3′, R 5′-GTG GAT TCA AGC ATA TCT CGG AA-3′), Pln (F 5′-AAA GTG CAA TAC CTC ACT CGC-3′, R 5′-GGC ATT TCA ATA GTG GAG GCT C-3′), Nppb (F 5′-GAG GTC ACT CCT ATC CTC TGG-3′, R G5′-CC ATT TCC TCC GAC TTT TCT C-3′). Western blot Samples were lysed and protein extracted according to the established protocols (Abcam). BCA (Biorad) was used to determine protein concentrations for loading. Samples were ran on 15% SDS–PAGE, transferred to nitrocellulose membranes and using the SNAP i.d. system (Millipore) probed with anti-ANP (Sigma, 1/500) or anti-β-actin (Millipore, 1/500) and anti-rabbit secondary antibody (Abcam). Development was by West Pico chemiluminescent substrate (Thermo Scientific) with 10 s exposure to autoradiography film. Band intensity was determined by ImageJ 1.47. Images have been cropped for presentation. Full-size images are presented in Supplementary Figs 18 and 19 . Statistical analysis Animal numbers were initially predetermined using Mead’s resource equation. Data were analysed using GraphPad Prism (GraphPad Software, CA) and are represented as the mean±s.e.m. Unpaired Student’s t -test was used to determine differences between two groups. P <0.05 was considered statistically significant. Outliers were determined and excluded using Grubb’s test. For human data, χ 2 -test was used to determine the difference between proportions, and Spearman’s rank correlation was used. To validate findings, each experiment was performed at least twice. Significance in microbiota comparisons was calculated with Qiime-based ANOVA, beta diversity significance was based on Anosim and 10 6 Monte Carlo permutations. Non-parametric two-sample t -test with 1000 Monte Carlo permutations was used in alpha diversity comparisons. Accession codes: Gene microarray data was deposited in GEO, accession number GSE69525 . How to cite this article: Thorburn, A. N. et al. Evidence that asthma is a developmental origin disease influenced by maternal diet and bacterial metabolites. Nat. Commun. 6:7320 doi: 10.1038/ncomms8320 (2015).